Structure of the hexameric HerA ATPase reveals a mechanism of translocation-coupled DNA-end processing in archaea The HerA ATPase cooperates with the NurA nuclease and the Mre11–Rad50 complex for the repair of double-strand DNA breaks in thermophilic archaea. Here we extend our structural knowledge of this minimal end-resection apparatus by presenting the first crystal structure of hexameric HerA. The full-length structure visualizes at atomic resolution the N-terminal HerA-ATP synthase domain and a conserved C-terminal extension, which acts as a physical brace between adjacent protomers. The brace also interacts in trans with nucleotide-binding residues of the neighbouring subunit. Our observations support a model in which the coaxial interaction of the HerA ring with the toroidal NurA dimer generates a continuous channel traversing the complex. HerA-driven translocation would propel the DNA towards the narrow annulus of NurA, leading to duplex melting and nucleolytic digestion. This system differs substantially from the bacterial end-resection paradigms. Our findings suggest a novel mode of DNA-end processing by this integrated archaeal helicase–nuclease machine. Ring-shaped helicases and translocases harness the chemical energy liberated from the hydrolysis of nucleotide triphosphate (NTP) and convert it into mechanical motion along DNA or RNA substrates, which they encircle [1] , [2] , [3] , [4] , [5] . The archaeal HerA and bacterial FtsK proteins are the founding members of a superfamily of ASCE (additional strand conserved E) RecA-like ATPases [6] with identified functions in chromosome segregation during cell division, conjugation or DNA repair events [7] . In addition, viral homologues in this clade are responsible for packaging genetic material into the capsid following replication [7] , [8] , [9] . Common to all ASCE-fold proteins, the nucleotide-binding site is formed at the junction between two protomers, and thus a hexameric complex will most commonly utilize six catalytic sites [10] . The major contribution to nucleotide binding is provided by highly conserved cis -acting amino acids (harboured within the classic Walker A and B motifs [11] ) located on the first subunit, while trans- acting elements donated from a second neighbouring subunit complete the site. These trans- acting residues are generally positively charged amino acids, and are often (but not exclusively) arginines, and thus commonly referred to as arginine fingers or sensors [10] , [12] ; their role is to enhance NTP binding and catalysis, and to stabilize multimeric assembly. In addition, these residues play key roles in communicating the occupancy of the NTP-binding site, and the hydrolysis state of the nucleotide, from one subunit to the next. In all thermophilic archaea, HerA is found clustered within an operon that also encodes for the NurA nuclease and the highly conserved Mre11 and Rad50 DNA repair proteins [7] , [13] , [14] , [15] , [16] , [17] . The HerA protein forms a strong physical association with NurA [16] , [18] , [19] and the resulting HerA–NurA complex is competent to digest double-stranded (ds)DNA substrates [14] , [16] , [19] . In eukaryotic organisms, the Mre11–Rad50 complex recognizes and binds to double-stranded breaks in the DNA, before recruiting specific helicase and nuclease components to promote repair by homologous recombination (HR) [20] , [21] , [22] . The integrated activity of these dedicated helicase–nuclease systems is responsible for DNA end-resection. This process generates the 3′ single-stranded tails that are then coated by the Rad51 recombinase, to initiate strand invasion and HR-driven DNA repair. The operonic linkage of HerA, NurA, Mre11 and Rad50 suggests that the HerA–NurA complex may play analogous roles to the eukaryotic helicase and nuclease components that work downstream of the Mre11–Rad50 complex, to perform the DNA end-resection in archaeal organisms [7] , [14] , [19] , [21] . To date, the emerging structural and biochemical evidence from archaeal systems is supportive of this concept [13] , [14] , [15] , [16] , [17] , [18] , [19] . In this study, we present the crystal structure of the HerA hexameric assembly from the thermophilic archaeon Sufolobus solfataricus , in complex with adenosine 5′—(β,γ-imido)triphosphate (AMP-PNP), a non-hydrolysable analogue of adenosine triphosphate (ATP). The HerA ring forms a toroid with an ~25-Å-wide central channel that is broad enough to accommodate B-form dsDNA. The hexameric assembly observed in the structure is stabilized by protrusions from both the N- and a C termini of each subunit, which embrace the neighbouring protomer to promote multimerization. Furthermore, while the C-terminal extension appears to be intrinsically linked to the catalytic nucleotide-binding site, the N-terminal appendage provides an exposed hydrophobic surface, which is crucial for NurA binding. Although the HerA hexamer appears ideally suited for translocating along a DNA duplex, the narrower annulus of the NurA dimer [16] , [18] likely acts as a ‘ploughshare’ [23] , [24] , resulting in separation of the DNA strands during archaeal DNA repair events. Combining structural and functional data, we propose a model for DNA translocation and processing by this putative archaeal DNA end-resection apparatus. Structure solution and architecture of the HerA hexamer Initial efforts to crystallize S. solfataricus HerA ( Sso 2251) yielded only poorly diffracting crystals. Two strategies were therefore employed, in combination, to improve crystal quality. The first was to mutate methionine residues 51 and 82 to leucine, to suppress an observed heterogeneity in start-codon usage. The second strategy involved the mutagenesis of solvent-exposed residues, such as lysine and glutamate, to minimize surface side-chain entropy and favour growth of well-ordered crystals. 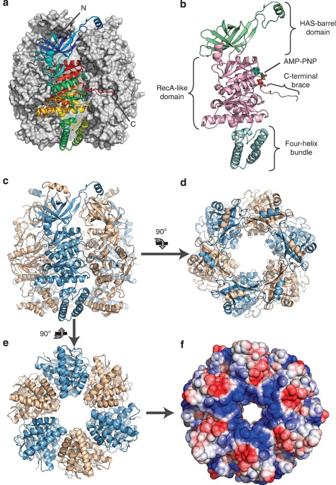Figure 1: Architecture of the HerA helicase. (a) Side view of the HerA hexamer generated by the threefold crystallographic symmetry of the R3:H spacegroup. The foremost protomer is drawn as a ribbon and coloured from the N- (blue) to the C-end (red), while the other five protomers are shown as a grey surface. (b) Side view of a monomer of HerA, coloured by domain, with the HAS barrel, ATPase and four-helix bundle domains in light green, light magenta and aquamarine, respectively. The bound AMP-PNP is represented by coloured sticks. (c) Side view of the HerA hexamer with protomers coloured alternatively in light blue and wheat. (d) Top-down view of the HerA hexamer. The HAS-barrel helical extensions embrace adjacent protomers. (e) Bottom-up view of the HerA hexamer. (f) Solvent-accessible surface representation ofe, coloured by electrostatic potential (±3 kT, blue/red). The positively charged entrance to the HerA hexameric pore appears well suited to accommodate dsDNA. All figures generated using PyMOL57; electrostatic surface calculated using APBS58and PDB ID 2PQR59. This HerA construct harboured a total of 10 amino-acid substitutions (HerAm10: full details are given in Supplementary Methods ; Supplementary Table 1 ), while retaining catalytic activity ( Supplementary Fig. 1 ). 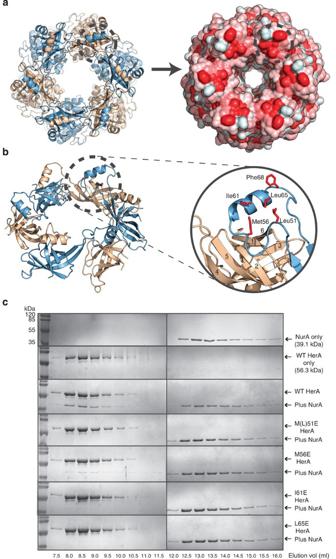Figure 2: A conserved hydrophobic patch on the HerA HAS-barrel mediates NurA binding. A helical extension from the N-terminal HAS- (HerA and ATP synthase) barrel domain embraces the neighbouring protomer and forms an exposed hydrophobic surface that interacts with the NurA nuclease. (a) A hydrophobic patch on the HerA HAS-barrel (dotted circle). Left: top-down view of the HerA hexamer (as shown inFig. 1d). Right: surface representation, identifying exposed hydrophobic surfaces, coloured in red. (b) Cartoon representation of the toroidal arrangement of β-barrel domains crowning the HerA hexameric assembly (view tilted fromaby 45°). A helical extension looping out between the 4th and 5th strands of the HAS-barrel domain is seen to embrace an adjacent barrel and form a hydrophobic patch (dotted circle). Inset: close-up cartoon representation of the HAS-barrel helical extension (in blue), with surface-exposed hydrophobic residues (M51, M56, I61, L65 and F68) shown as red sticks. β-strands of the adjacent barrel (in wheat) are numbered 1 through to 6. Figures generated using PyMOL57. (c) Characterization of the NurA interaction surface of HerA. Gel filtration analysis of HerA–NurA complex formation, examining the interaction of NurA with either native HerA, or four individual HerA point mutations of residues exposed on the hydrophobic surface (M51E, M56E, I61E and L65E). Fractions eluted from the S200 HR 10/300 gel filtration column were resolved by SDS–polyacrylamide gel electrophoresis. Chromatography ultraviolet traces for all elution profiles are displayed inSupplementary Fig. 3. The HerAm10 protein yielded highly diffracting crystals that were used to determine the X-ray structure of HerA at 2.85 Å (PDB ID 4D2I; data collection and refinement statistics given in Supplementary Table 2 ). Full-length HerAm10 crystallized in spacegroup R3:H, with two protomers in the asymmetric unit, each bound to one AMP-PNP molecule ( Supplementary Fig. 2a,c ). The hexameric ring, considered as the functionally relevant oligomeric assembly of HerA, is generated by the threefold crystallographic symmetry ( Fig. 1a,c–f ). Overall, the HerA ring has a compact architecture with dimensions of ~100 Å across and ~100 Å in height; a central channel of ~25 Å in diameter is well suited for accommodating approximately three turns of B-form dsDNA. The entire chain of the HerA protomer was visible in the electron density map, with the exclusion of 23 amino acids at the C terminus, which were disordered. Thus, our crystallographic model visualizes all three domains of the HerA protomer: the N-terminal β-barrel domain, the central RecA-like catalytic core and a flanking four-helix bundle ( Fig. 1b ). The tripartite structure of the HerA protomer adopts an extended conformation, so that each domain of the protomer makes extensive interactions with the same domain of adjacent chains in the hexameric ring. The four-helix bundles arrange to form the putative entrance to the pore, providing a positively charged surface suitable for guiding DNA into the channel ( Fig. 1e,f ). Structural homology searches using the PDBeFold SSM server ( http://www.ebi.ac.uk/msd-srv/ssm/ ) identified Thermoanaerobacter pseudethanolicus VirB4 (an ATPase of the bacterial Type IV secretion system) as the closest structural homologue of HerA (PDB ID 4AG5 (ref. 25 ), with an r.m.s.d. of 2.9 Å over 275 Cα atoms of the RecA-like and helix bundle domains; Supplementary Fig. 2b ). Figure 1: Architecture of the HerA helicase. ( a ) Side view of the HerA hexamer generated by the threefold crystallographic symmetry of the R3:H spacegroup. The foremost protomer is drawn as a ribbon and coloured from the N- (blue) to the C-end (red), while the other five protomers are shown as a grey surface. ( b ) Side view of a monomer of HerA, coloured by domain, with the HAS barrel, ATPase and four-helix bundle domains in light green, light magenta and aquamarine, respectively. The bound AMP-PNP is represented by coloured sticks. ( c ) Side view of the HerA hexamer with protomers coloured alternatively in light blue and wheat. ( d ) Top-down view of the HerA hexamer. The HAS-barrel helical extensions embrace adjacent protomers. ( e ) Bottom-up view of the HerA hexamer. ( f ) Solvent-accessible surface representation of e , coloured by electrostatic potential (±3 kT, blue/red). The positively charged entrance to the HerA hexameric pore appears well suited to accommodate dsDNA. All figures generated using PyMOL [57] ; electrostatic surface calculated using APBS [58] and PDB ID 2PQR [59] . Full size image In agreement with earlier bioinformatic predictions [7] the first 104 amino acids of the HerA protein form a six-stranded β-barrel domain (absent from the VirB4 protomer; Supplementary Fig. 2b ), which bears clear similarity to the β-barrel fold seen at the N terminus of the bovine F 1 -ATP synthase [26] , PDB ID 1BMF). The HerA HAS (HerA and ATP synthase [7] ) β-barrel domains form an N-terminal toroidal crown, assembled on top of the central hexameric ring of RecA-like domains. Uniquely to the HAS domain of HerA, a helical extension originating between the 4th and 5th strands of each β-barrel ( Figs 1a–d and 2a,b ) packs against the top of the adjacent HAS barrel, apparently stabilizing the hexameric assembly. Figure 2: A conserved hydrophobic patch on the HerA HAS-barrel mediates NurA binding. A helical extension from the N-terminal HAS- (HerA and ATP synthase) barrel domain embraces the neighbouring protomer and forms an exposed hydrophobic surface that interacts with the NurA nuclease. ( a ) A hydrophobic patch on the HerA HAS-barrel (dotted circle). Left: top-down view of the HerA hexamer (as shown in Fig. 1d ). Right: surface representation, identifying exposed hydrophobic surfaces, coloured in red. ( b ) Cartoon representation of the toroidal arrangement of β-barrel domains crowning the HerA hexameric assembly (view tilted from a by 45°). A helical extension looping out between the 4th and 5th strands of the HAS-barrel domain is seen to embrace an adjacent barrel and form a hydrophobic patch (dotted circle). Inset: close-up cartoon representation of the HAS-barrel helical extension (in blue), with surface-exposed hydrophobic residues (M51, M56, I61, L65 and F68) shown as red sticks. β-strands of the adjacent barrel (in wheat) are numbered 1 through to 6. Figures generated using PyMOL [57] . ( c ) Characterization of the NurA interaction surface of HerA. Gel filtration analysis of HerA–NurA complex formation, examining the interaction of NurA with either native HerA, or four individual HerA point mutations of residues exposed on the hydrophobic surface (M51E, M56E, I61E and L65E). Fractions eluted from the S200 HR 10/300 gel filtration column were resolved by SDS–polyacrylamide gel electrophoresis. Chromatography ultraviolet traces for all elution profiles are displayed in Supplementary Fig. 3 . Full size image While the extension from the HAS domain fastens the N-terminal crown of the assembly, a C-terminal protrusion also stabilizes the hexamer by traversing the nucleotide-binding site to embrace the RecA-like domain of the neighbouring protomer ( Fig. 1a,b ). Thus, protrusions from both the N- and C termini engage in inter-subunit contacts that contribute to stabilizing the multimeric assembly ( Fig. 1a–d ). In addition, the C-terminal extension associates with the catalytic nucleotide-binding site of the neighbouring subunit; this critical interaction is discussed in detail below. The HAS domain mediates the interaction with NurA Inspection of the protomer-bridging α-helical extension at the top of the HAS barrel revealed a hydrophobic patch formed by residues L51 (mutated from M51 in the HerAm10), M56, I61 and L65 ( Fig. 2a,b ). As we had previously established that the HAS domain was crucial for the interaction with the NurA nuclease [16] , we reasoned that this exposed hydrophobic site might mediate the association with NurA. We therefore performed site-directed mutagenesis of these four hydrophobic residues, reversing their chemical nature by mutation to the charged residue glutamic acid. As predicted, the individual mutations resulted in a significantly weakened interaction with NurA, as determined by analytical gel filtration chromatography ( Fig. 2c ; Supplementary Fig. 3 ). Thus, we propose that the α-helical extension of the HAS domain performs two essential and complementary roles, by providing an exposed hydrophobic surface for interaction with NurA, and stabilizing the hexameric assembly by homotypic in trans interaction with the HAS barrel of the adjacent subunit. The C-terminal ‘brace’ interacts with the ATP-binding site The RecA-like ATPase domain is located in the middle of the HerA protomer and consists of a central seven-strand parallel β-sheet surrounded by eight α-helices ( Fig. 1b ). The β-sheet terminates with four additional antiparallel strands [7] , [27] , folded as a separate, distorted sheet-like structure. Extending from this feature, the aforementioned C-terminal protrusion traverses the active site to embrace the adjacent protomer ( Fig. 3a ). 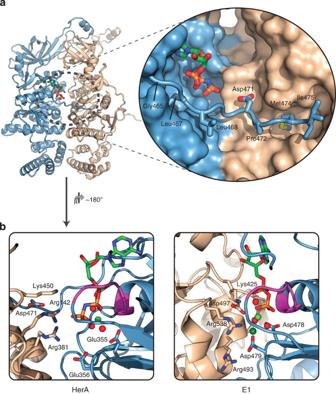Figure 3: A C-terminal brace associates with the ATP-binding site. (a) Left: cartoon representation of the two HerA protomers present in the asymmetric unit. Chain A is coloured light blue; chain B is coloured wheat. Bound AMP-PNP (stick representation) is located at the interface between protomers. Right (inset): close-up surface representation of the interface between the protomers, with the bound AMP-PNP shown as sticks. A flexible C-terminal brace from chain A shown in cartoon format extends across the active site to embrace chain B. Hydrophobic residues G465, L467, L468, P472, M474 and I475 (shown as sticks) position the brace. The acidic residue D471 protrudes towards the active site. (b) Cartoon comparison of the HerA active site with that of the E1 helicase (PDB id 2GXA) in an ATP-type conformation. Left: HerA active site between chains A (light blue) and B (wheat), viewed from inside the DNA-binding pore, with bound AMP-PNP and key residues shown as sticks. Bound magnesium and water moieties shown as pale green and red spheres, respectively. Chain A donates the Walker A motif (magenta; sticks omitted), and Walker B motif (E355 and E356). Chain B donates three positively charged residues (from the top, K450, R142 and R381). R381 forms a salt bridge with Walker B glutamate E356, while R142 directly interacts with the γ-phosphate of the ATP-mimic. The conserved acidic brace residue (D471) forms a salt bridge with R142, positioning this arginine at the active site. Right: comparative view of the E1 ‘ATP-type’ active site between Chains A (light blue) and B (wheat). Key residues and bound ADP shown as sticks. Bound magnesium and water moieties shown as pale green and red spheres, respectively, and bound chloride (mimicking ATP γ-phosphate) as a dark-green sphere. As in HerA, chain A donates the Walker A motif (magenta) and Walker B aspartates (D478 and D479), while chain B donates three positively charged residues (from the top, K425, R538 and R493). Acis-acting aspartate (D497) interacts with the middle of these residues, in a manner similar to the R142/D471 interaction in HerA. All figures are generated using PyMOL57. Figure 3: A C-terminal brace associates with the ATP-binding site. ( a ) Left: cartoon representation of the two HerA protomers present in the asymmetric unit. Chain A is coloured light blue; chain B is coloured wheat. Bound AMP-PNP (stick representation) is located at the interface between protomers. Right (inset): close-up surface representation of the interface between the protomers, with the bound AMP-PNP shown as sticks. A flexible C-terminal brace from chain A shown in cartoon format extends across the active site to embrace chain B. Hydrophobic residues G465, L467, L468, P472, M474 and I475 (shown as sticks) position the brace. The acidic residue D471 protrudes towards the active site. ( b ) Cartoon comparison of the HerA active site with that of the E1 helicase (PDB id 2GXA) in an ATP-type conformation. Left: HerA active site between chains A (light blue) and B (wheat), viewed from inside the DNA-binding pore, with bound AMP-PNP and key residues shown as sticks. Bound magnesium and water moieties shown as pale green and red spheres, respectively. Chain A donates the Walker A motif (magenta; sticks omitted), and Walker B motif (E355 and E356). Chain B donates three positively charged residues (from the top, K450, R142 and R381). R381 forms a salt bridge with Walker B glutamate E356, while R142 directly interacts with the γ-phosphate of the ATP-mimic. The conserved acidic brace residue (D471) forms a salt bridge with R142, positioning this arginine at the active site. Right: comparative view of the E1 ‘ATP-type’ active site between Chains A (light blue) and B (wheat). Key residues and bound ADP shown as sticks. Bound magnesium and water moieties shown as pale green and red spheres, respectively, and bound chloride (mimicking ATP γ-phosphate) as a dark-green sphere. As in HerA, chain A donates the Walker A motif (magenta) and Walker B aspartates (D478 and D479), while chain B donates three positively charged residues (from the top, K425, R538 and R493). A cis -acting aspartate (D497) interacts with the middle of these residues, in a manner similar to the R142/D471 interaction in HerA. All figures are generated using PyMOL [57] . Full size image A similar protrusion (referred to as a ‘brace’) has previously been shown to stabilize hexameric assembly in the E1 papillomavirus replicative helicase [28] . Indeed, a basic model of this E1 brace was also proposed, based on small-angle X-ray scattering (SAXS) measurements [28] . Our crystallographic analysis provides a view of the HerA brace at atomic resolution, revealing novel features. A series of conserved hydrophobic contacts keeps the brace pinned to the two HerA protomers, while a conserved glycine residue (G465) provides flexibility to the arrangement ( Fig. 3a ). The hydrophobic positioning of the brace helps orient a conserved aspartate (D471) towards the nucleotide-binding site, at the cleft between protomers ( Fig. 3a ). Structural superposition of the nucleotide-binding sites of both the HerA and E1 proteins revealed further interesting similarities ( Fig. 3b ). Although E1 belongs to the AAA+, rather than the RecA-like family of ATPases [29] , [30] , the arrangement of catalytic residues surrounding the nucleotide-binding cleft is comparable in E1 and HerA ( Fig. 3b and PDB ID 2GXA [31] ). Since the E1 ring-shaped ATPase represents a paradigm for DNA translocation, we decided to explore potential mechanistic similarities between these two proteins. The structural superposition of HerA and E1 revealed conservation of the key cis -acting residues that form the P-loop (ATP phosphate group-binding loop) of the Walker A motif, and the acidic catalytic elements of the Walker B motif on the first subunit. In addition, three basic residues donated in trans from the neighbouring subunit are also conserved in the E1 and HerA structures ( Fig. 3b ). In all ring-shaped ASCE ATPases, trans -acting residues facilitate catalysis by stabilizing the transition state during nucleotide hydrolysis [1] , [3] , [10] , [12] . In both the HerA and E1 structures, the middle of the three basic trans -acting residues (R142 and R538, respectively) associates with the nucleotide γ-phosphate mimic ( Fig. 3b ), apparently positioning it for nucleophilic attack. In the AMP-PNP-bound state observed in the HerA structure, the second trans -acting arginine, R381, forms a salt bridge with E356 of the Walker B motif. This interaction is deemed necessary for both stable interface formation and water activation prior to catalysis [1] . Intriguingly, in the HerA structure the R142 trans -acting residue also forms a salt bridge with the previously described aspartate D471 ( Fig. 3b ), harboured on the C-terminal brace of the neighbouring protomer ( Fig. 3a,b ). A similar acidic residue (D497) interacts with the equivalent arginine in the E1 structure (R538), although this aspartate acts in -cis from the same chain ( Fig. 3b ). Nevertheless, the equivalent arrangement of these acidic residues at the nucleotide-binding sites of both enzymes suggests a common function. Since the HerA brace interacts with the R142 trans -acting residue of the adjacent protomer at the nucleotide-binding cleft, it seems plausible that this extension also plays important functional roles in the chemo-mechanical cycle. Mutational analysis of the nucleotide-binding site Having identified the key amino acids conserved at the ATP-binding site of HerA, we performed site-directed mutagenesis to examine their role in catalysis. We mutated the P-loop lysine of the Walker A motif (K154A), the trans -acting arginine residues (R142A and R381A) and the aspartate 471 on the C-terminal brace (D471A), switching to alanine in each case. Three different functional assays were employed to investigate the effect of these substitutions: an ATPase assay ( Fig. 4a ), to measure ATP hydrolysis by the wild-type (WT) and mutant HerA–NurA complexes [16] ; a DNA destruction assay ( Fig. 4b ; Supplementary Fig. 4 ), to examine the ability of the HerA–NurA complex to translocate and digest a linear 5.3-kb dsDNA substrate; and a DNA-unwinding assay by a nuclease-inactivated HerA–D58A NurA complex, using short radiolabelled oligonucleotide substrates ( Fig. 4c ; Supplementary Fig. 5 ), as described in our previous study [16] . 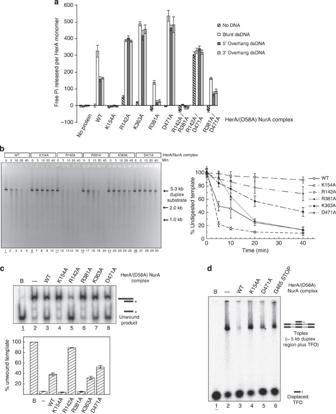Figure 4: Functional assays examining ATP hydrolysis and DNA processing by HerA–NurA. (a) ATPase assays measuring free Pirelease by the HerA–(D58A) NurA complex. Three DNA substrates were used: blunt-ended dsDNA, or dsDNA with 5′ or 3′ single-stranded tails, respectively. Native HerA (WT), the Walker A mutant (K154A), thetrans-acting arginine mutants (R142A and R381A), the putative DNA-binding loop mutant (K363A), the ‘brace’ mutation (D471A) and the R142A/R381A, R142A/D471A and R381A/D471A mutants were examined. The data points represent the mean of three independent repeats and the error bars one s.d. (b) (Left) DNA-processing assays of a 5.3-kb dsDNA substrate (using 2 μM of the HerA–NurA complex on 1.25 nM dsDNA at 60 °C). Products were examined at five time points: 0 (underlined), 5, 10, 20 and 40 min, following separation on a 0.8% agarose gel and visualization by ethidium bromide staining. Lanes 1–5, WT HerA–WT NurA complex; lanes 6–10, K154A HerA–WT NurA; lanes 11–15, R142A HerA–WT NurA; lanes 16–20, R381A HerA–WT NurA; lanes 21–25, K363A HerA–WT NurA; lanes 26–30, D471A HerA–WT NurA. (Right) assay quantification. The data points represent the mean of three independent repeats and the error bars one s.d. Additional controls are shown inSupplementary Fig. 4. (c) (Top) DNA-unwinding activity by HerA–(D58A) NurA (0.46 μM HerA–NurA complex and 10 nM dsDNA, 5′ single-stranded overhanging, substrate)16. After 30 min at 60 °C, products were resolved by 12% polyacrylamide gel electrophoresis and visualized by autoradiography. The DNA was32P radiolabelled on the 5′ end of the shorter strand (asterisk). Lane 1 (underlined), boiled (unwound) sample; lane 2, no protein control; lanes 3–8, native (WT) HerA, and K154A, R142A, R381A, K363A and D471A mutant HerA, respectively (all in complex with D58A NurA). (Bottom) assay quantification. The data points represent the mean of three independent repeats and the error bars one s.d. (d) Triplex displacement assay. Lane 1 (underlined) boiled control (TFO;32P radiolabelled triplex-forming oligonucleotide (asterisk)); lane 2, no protein control; lanes 3–6, native (WT) HerA, and K154A, D471A and G465STOP mutant HerA, respectively (all in complex with D58A NurA). Products were resolved on a 1% agarose gel, and visualized by autoradiography. Figure 4: Functional assays examining ATP hydrolysis and DNA processing by HerA–NurA. ( a ) ATPase assays measuring free P i release by the HerA–(D58A) NurA complex. Three DNA substrates were used: blunt-ended dsDNA, or dsDNA with 5′ or 3′ single-stranded tails, respectively. Native HerA (WT), the Walker A mutant (K154A), the trans -acting arginine mutants (R142A and R381A), the putative DNA-binding loop mutant (K363A), the ‘brace’ mutation (D471A) and the R142A/R381A, R142A/D471A and R381A/D471A mutants were examined. The data points represent the mean of three independent repeats and the error bars one s.d. ( b ) (Left) DNA-processing assays of a 5.3-kb dsDNA substrate (using 2 μM of the HerA–NurA complex on 1.25 nM dsDNA at 60 °C). Products were examined at five time points: 0 (underlined), 5, 10, 20 and 40 min, following separation on a 0.8% agarose gel and visualization by ethidium bromide staining. Lanes 1–5, WT HerA–WT NurA complex; lanes 6–10, K154A HerA–WT NurA; lanes 11–15, R142A HerA–WT NurA; lanes 16–20, R381A HerA–WT NurA; lanes 21–25, K363A HerA–WT NurA; lanes 26–30, D471A HerA–WT NurA. (Right) assay quantification. The data points represent the mean of three independent repeats and the error bars one s.d. Additional controls are shown in Supplementary Fig. 4 . ( c ) (Top) DNA-unwinding activity by HerA–(D58A) NurA (0.46 μM HerA–NurA complex and 10 nM dsDNA, 5′ single-stranded overhanging, substrate) [16] . After 30 min at 60 °C, products were resolved by 12% polyacrylamide gel electrophoresis and visualized by autoradiography. The DNA was 32 P radiolabelled on the 5′ end of the shorter strand (asterisk). Lane 1 (underlined), boiled (unwound) sample; lane 2, no protein control; lanes 3–8, native (WT) HerA, and K154A, R142A, R381A, K363A and D471A mutant HerA, respectively (all in complex with D58A NurA). (Bottom) assay quantification. The data points represent the mean of three independent repeats and the error bars one s.d. ( d ) Triplex displacement assay. Lane 1 (underlined) boiled control (TFO; 32 P radiolabelled triplex-forming oligonucleotide (asterisk)); lane 2, no protein control; lanes 3–6, native (WT) HerA, and K154A, D471A and G465STOP mutant HerA, respectively (all in complex with D58A NurA). Products were resolved on a 1% agarose gel, and visualized by autoradiography. Full size image We had previously shown that NurA association was required for HerA catalytic activity [16] , and therefore the HerA–NurA complex was used in all three assays. Consistent with our previous work [16] , the WT complex displayed an approximately twofold higher level of ATPase activity on blunt- relative to overhang dsDNA substrates ( Fig. 4a ). Furthermore, no activity was detectable in the absence of the DNA substrate, in keeping with our previous results [16] . In addition, the K154A Walker A mutation [11] resulted in the complete loss of activity in all functional assays, as expected ( Fig. 4a ; Fig. 4b , lanes 6–10; Fig. 4c , lane 4). In contrast, mutation of the R142 trans -acting residue generated unanticipated results. The proximity of this residue to the terminal phosphate of the AMP-PNP in the structure was indicative of a role in catalysis; similar arrangements in other multimeric ATPases have been proposed to stabilize the transition state during nucleotide hydrolysis [1] . However, rather than inhibiting the complex, the R142A mutation appeared to stimulate the catalytic activity of the HerA–NurA complex ( Fig. 4a ; Fig. 4b , lanes 11–15; Fig. 4c , lane 5). The most notable effect was observed in the ATPase assay: while activity increased relative to the WT complex for all three DNA substrates, stimulation was most pronounced on the substrates with overhangs ( Fig. 4a ). Thus, while the WT complex processed blunt-ended substrates more efficiently than those with overhangs, this difference was not observed in the R142A mutant, and a similar high level of ATPase activity was seen on both types of substrate. Intriguingly, the R142A mutation also resulted in a subtle increase in ATPase activity in the absence of a DNA substrate. Taken together, these observations suggest that the R142 residue performs a more regulatory function in the chemo-mechanical cycle of the HerA–NurA complex, rather than a lead role in catalysis. In contrast, the R381A mutation had an inhibitory effect on the activity of the complex, but to a different extent in the various assays. Thus, the R381A HerA mutant complex was incapable of DNA unwinding ( Fig. 4c , lane 6) and its ATPase activity was severely impaired, while its activity in the DNA destruction assay was also reduced, but not abrogated ( Fig. 4a ; Fig. 4b , lanes 16–20). Intriguingly, R381 did not interact directly with the AMP-PNP moiety in the crystal structure, suggesting a possible conformational reconfiguration of the ATP-binding site during catalysis. Indeed, sequence alignments of HerA with other hexameric RecA-like helicases revealed that the R381 residue is equivalent to the arginine finger residue of TrwB (R375), VirB4 (R496) and FtsK (R620) ( Fig. 5 ) [7] , [25] , [32] , [33] , [34] . In both TrwB and VirB4 this trans -acting arginine residue has been shown to be mobile, positioning at the nucleotide-binding site to interact with the ATP terminal phosphate during hydrolysis [25] , [32] . Taken together, the results of the functional assays for R142 and R381 suggest a partial functional redundancy between the two trans -acting arginines. Indeed, a complete loss of ATPase activity was only observed with a double alanine mutation of both arginines, R142A/R381A ( Fig. 4a ). 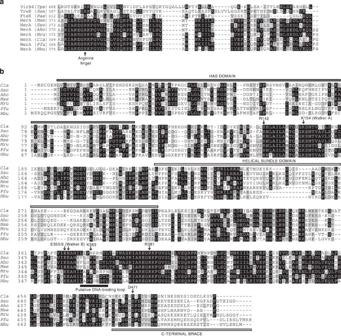Figure 5: Sequence conservation of HerA residues important for nucleotide binding and hydrolysis, and DNA translocation. (a) Conservation of the arginine finger residue in the HerA-FtsK superfamily of proteins. Multiple sequence alignment of archaeal HerA amino-acid sequences (Cla,Caldisphaera lagunensis;Sso,Sulfolobus solfataricus;Aho,Acidianus hospitalis;Mse,Metallosphaera sedula;Mru,Methanobrevibacter ruminantium;Pfu,Pyrococcus furiosus;Hbu,Hyperthermus butylicus) alongside the closely related proteins TrwB (Sen,Salmonella enterica), FtsK (Pae,Pseudomonas aeruginosa) and VirB4 (Tps,Thermoanaerobacter pseudethanolicus). InS. solfataricusHerA this residue is R381 (ref.7); inP. aeruginosaFtsK, R620 (refs7,34); inS. entericaTrwB, R375 (refs7,31) and inT. pseudethanolicusVirB4, R496 (refs7,25,33). Identically conserved residues are shaded in black, and partially conserved residues in grey. (b) Alignment of the five full-length archaeal HerA sequences shown ina. TheSsoWalker A lysine (K154),trans-acting arginines (R142 and R381), DNA-binding loop lysines (K363 and K395) and the C-terminal brace aspartate (D471) are indicated with arrows. The grey box above the N-terminal sequences denotes the HAS-barrel domain, while the helical-bundle domain is indicated by a white box. The light grey box below the C-terminal sequences indicates the C-terminal brace, while the black box under the sequences centred atSsoK363 denotes the putative DNA-binding loop. In all species, the gene encoding the HerA protein is encompassed within an archaeal DNA end-resection operon, which also harbours the NurA, Mre11 and Rad50 genes. Figure 5: Sequence conservation of HerA residues important for nucleotide binding and hydrolysis, and DNA translocation. ( a ) Conservation of the arginine finger residue in the HerA-FtsK superfamily of proteins. Multiple sequence alignment of archaeal HerA amino-acid sequences ( Cla , Caldisphaera lagunensis ; Sso , Sulfolobus solfataricus ; Aho , Acidianus hospitalis ; Mse , Metallosphaera sedula ; Mru , Methanobrevibacter ruminantium ; Pfu , Pyrococcus furiosus ; Hbu , Hyperthermus butylicus ) alongside the closely related proteins TrwB ( Sen , Salmonella enterica ), FtsK ( Pae , Pseudomonas aeruginosa ) and VirB4 ( Tps , Thermoanaerobacter pseudethanolicus ). In S. solfataricus HerA this residue is R381 (ref. 7 ); in P. aeruginosa FtsK, R620 (refs 7 , 34 ); in S. enterica TrwB, R375 (refs 7 , 31 ) and in T. pseudethanolicus VirB4, R496 (refs 7 , 25 , 33 ). Identically conserved residues are shaded in black, and partially conserved residues in grey. ( b ) Alignment of the five full-length archaeal HerA sequences shown in a . The Sso Walker A lysine (K154), trans -acting arginines (R142 and R381), DNA-binding loop lysines (K363 and K395) and the C-terminal brace aspartate (D471) are indicated with arrows. The grey box above the N-terminal sequences denotes the HAS-barrel domain, while the helical-bundle domain is indicated by a white box. The light grey box below the C-terminal sequences indicates the C-terminal brace, while the black box under the sequences centred at Sso K363 denotes the putative DNA-binding loop. In all species, the gene encoding the HerA protein is encompassed within an archaeal DNA end-resection operon, which also harbours the NurA, Mre11 and Rad50 genes. Full size image The brace influences the catalytic activity of HerA–NurA The direct interaction of the C-terminal brace with trans -acting R142 prompted us to investigate its role in the activity of the HerA–NurA complex. Alanine mutation of the conserved D471 caused a severe impairment in the DNA destruction assays ( Fig. 4b , lanes 26–30). In addition, a triplex displacement assay, which specifically measured the ability of the complex to translocate on dsDNA and sterically exclude a Hoogstein-bonded triplex strand [16] , [35] , confirmed that the D471A mutant resulted in reduced levels of DNA translocation ( Fig. 4d , lane 5). Furthermore, premature truncation of the C-terminal tail by introduction of a stop codon at G465 produced a more severe inhibition ( Fig. 4d , lane 6). In contrast, ATPase activity increased as a result of the D471A mutation on all dsDNA substrates ( Fig. 4a ), with a most pronounced enhancement on the substrates with overhangs. Consequently, the resultant level of ATPase activity was now similar on all of the DNA substrates, as was observed with the R142A mutant ( Fig. 4a ). These data suggest that the D471 residue on the C-terminal brace is not required for the hydrolysis of ATP per se , but instead seems to assist in the conversion of ATP hydrolysis into DNA translocation. The roles of D471 and R142 in ATP hydrolysis were investigated further by generating a R142A/D471A double mutant. Whereas the WT complex required engagement of a DNA substrate for the activation of nucleotide hydrolysis, the ATPase activity of the R142A/D471A double mutant became independent of DNA. This substrate-independent ATP turnover was comparable to the activity observed with the WT complex on blunt-ended DNA ( Fig. 4a ). Thus, the DNA dependence of ATP hydrolysis observed in the WT complex appears to be mediated by interaction between R142 and D471. In contrast, a HerA–NurA complex containing the double R381A/D471A HerA mutant was completely inactive in the absence of a DNA substrate ( Fig. 4a ). We noted, however, that DNA substrates with single-stranded overhangs elicited a small rise in ATPase activity in this double mutant, relative to the R381A single mutant. Taken together, the results of the functional analysis suggest that the C-terminal brace of HerA has an important yet complex role in coupling ATP hydrolysis to mechanical work. A putative DNA-binding loop is linked to the active site In hexameric ATPases, the concerted movement of pore-lining DNA-binding loops has been shown to drive translocation along DNA substrates [31] , [36] , [37] . Closer inspection of the channel in the HerA ring revealed the presence of a loop spanning residues F360 to L368 and lining the inner surface of the central pore. The loop was located at the opposite end of the kinked α-helix bearing the trans -acting R381 residue ( Fig. 6a,b ). Alanine mutation of the conserved loop residue K363, which projects into the central pore [38] , resulted in impaired DNA processing in the destruction assays, and inhibition was also observed in the helicase assays ( Fig. 4b , lanes 21–25; Fig. 4c , lane 7). Conversely, ATPase activity actually increased in the K363A mutant, particularly on the substrates with single-stranded overhangs, as we observed with the R142A and D471A mutants ( Fig. 4a ). The partial uncoupling of ATP hydrolysis from mechanical work appears consistent with a role for K363 in DNA translocation. 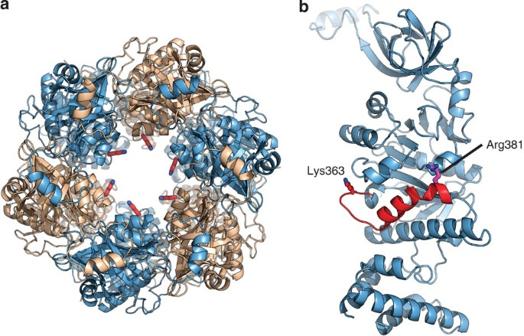Figure 6: A conserved DNA-binding loop appears mechanically linked to the active site. Each protomer of the HerA hexamer donates a conserved putative DNA-binding residue (K363) that protrudes into the DNA-binding channel from a flexible loop. (a) Left: top-down view of the HerA hexamer, with chain A protomers coloured light blue and chain B protomers coloured wheat (as shown inFig. 1d). DNA-binding K363 residues (red sticks) are seen protruding into the central channel. (b) Cartoon representation of chain A highlighting the putative DNA-binding loop, harbouring K363 (red stick). This lysine extends from the distorted helix (red) that also presents the key catalytic residue R381 (magenta stick) to the active site. All figures are generated using PyMOL57. Figure 6: A conserved DNA-binding loop appears mechanically linked to the active site. Each protomer of the HerA hexamer donates a conserved putative DNA-binding residue (K363) that protrudes into the DNA-binding channel from a flexible loop. ( a ) Left: top-down view of the HerA hexamer, with chain A protomers coloured light blue and chain B protomers coloured wheat (as shown in Fig. 1d ). DNA-binding K363 residues (red sticks) are seen protruding into the central channel. ( b ) Cartoon representation of chain A highlighting the putative DNA-binding loop, harbouring K363 (red stick). This lysine extends from the distorted helix (red) that also presents the key catalytic residue R381 (magenta stick) to the active site. All figures are generated using PyMOL [57] . Full size image The order of ATP hydrolysis events around the HerA ring We also investigated whether the sequence of ATP hydrolysis at the six nucleotide-binding sites of the hexameric ring followed an ordered and sequential pattern of events during translocation of the HerA–NurA complex along the DNA, as in previously published models of other multimeric helicases [31] , [37] , [39] , [40] . A mutant-doping approach, as described in previous studies [34] , [41] , [42] , was adopted, where the WT HerA protein was mixed with the catalytically inactive K154A mutant, resulting in the formation of heterologous HerA rings ( Supplementary Fig. 6 ). We followed the effect of K154A doping using the DNA-unwinding assay. Increasing the ratio of K154A to WT HerA resulted in an exponential drop in the proportion of unwound DNA substrate ( Fig. 7a,b ). This result indicated that the introduction of a single mutant subunit within the HerA ring rendered the complex incompetent for DNA unwinding. Thus, productive unwinding of DNA substrates requires a coordinated series of ATP hydrolysis events around the active sites of the HerA ring, as has been reported for other hexameric ATPases [34] , [41] , [42] . 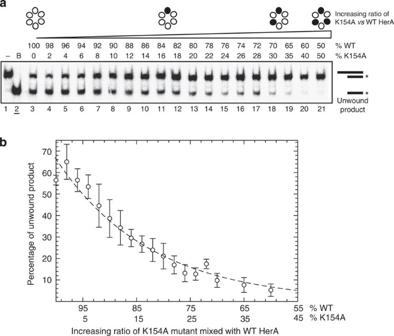Figure 7: Mutant-doping assays to examine the ordering of catalytic events around the hexameric ring. (a) Mutant doping with the K154A HerA in a DNA-unwinding assay. Lane 1, no protein control; lane 2 (underlined), boiled (unwound) control; lanes 3–21, native (WT) HerA and an increasing proportion of K154A HerA (0–50% K154A in 2% increments, respectively). The HerA proteins were mixed at 60 °C, prior to the addition of D58A (nuclease inactivated) NurA at 60 °C to form the HerA–NurA complex. After addition of the DNA substrate (32P radiolabeled on one strand, as denoted by the asterisk) the reactions were terminated after 30 min at 60 °C by the addition of SDS and EDTA. Products were resolved by 12% polyacrylamide gel electrophoresis and visualized by phosphoimaging. (b) Quantification and fitting of the mutant-doping data in the unwinding assays shown ina. The data points represent the mean of three independent repeats and the error bars one s.d. The data were fitted to a first-order exponential decay model using ‘ProFit’ software (www.quansoft.com). Figure 7: Mutant-doping assays to examine the ordering of catalytic events around the hexameric ring. ( a ) Mutant doping with the K154A HerA in a DNA-unwinding assay. Lane 1, no protein control; lane 2 (underlined), boiled (unwound) control; lanes 3–21, native (WT) HerA and an increasing proportion of K154A HerA (0–50% K154A in 2% increments, respectively). The HerA proteins were mixed at 60 °C, prior to the addition of D58A (nuclease inactivated) NurA at 60 °C to form the HerA–NurA complex. After addition of the DNA substrate ( 32 P radiolabeled on one strand, as denoted by the asterisk) the reactions were terminated after 30 min at 60 °C by the addition of SDS and EDTA. Products were resolved by 12% polyacrylamide gel electrophoresis and visualized by phosphoimaging. ( b ) Quantification and fitting of the mutant-doping data in the unwinding assays shown in a . The data points represent the mean of three independent repeats and the error bars one s.d. The data were fitted to a first-order exponential decay model using ‘ProFit’ software ( www.quansoft.com ). Full size image Small-angle X-ray scattering analysis of the HerA–NurA complex The structure-based mutagenesis data presented here are in agreement with the coaxial arrangement for the HerA–NurA complex predicted in our previously published study [16] , where the NurA dimer docks on top of the HAS-barrel face of the HerA hexamer. We note that the exposed hydrophobic patches on the surface of NurA [16] and HerA, identified by mutagenesis, appear suitably aligned to mediate this interaction ( Supplementary Fig. 7 ). To provide further insight into the mechanism of DNA-end processing by the HerA–NurA complex, we analysed its three-dimensional architecture by SAXS. SAXS analysis of the HerA–NurA complex resulted in the generation of a molecular envelope that is compatible with the predicted coaxial arrangement of the individual HerA and NurA components (see Fig. 8a ). Closer inspection of the envelope confirmed a pore-like cavity in the density, permitting unambiguous docking of the hexameric HerA crystal structure (see Fig. 8b ). Combining this observation with knowledge of the reciprocal hydrophobic interaction surfaces on HerA and NurA enabled subsequent docking of the dimeric NurA crystal structure [16] into the remaining density. SAXS data processing and model-generation steps are summarized in Fig. 8c–f , and full details of the experimental procedures and data analyses are provided in the Methods section. 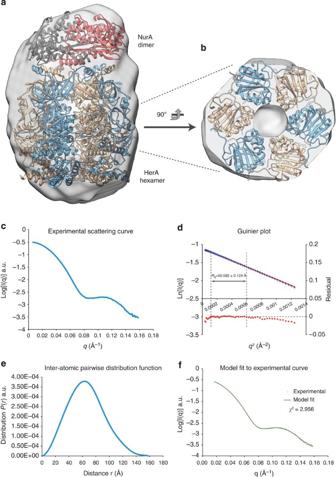Figure 8: SAXS analysis of the HerA–NurA complex. (a) and (b) lateral and axial views, respectively, of the molecular envelope generated byab initioSAXS modelling, with crystallographic models of HerA (PDB code: 4D2I) and NurA (PDB code: 2YGK) manually docked in it. The axial view is clipped at the level of the ATPase domains of the HerA hexamer, to visualize the pore-like cavity present in the SAXS envelope, which defines the position of HerA within the map. (c) Experimental SAXS curve for the HerA–NurA complex, in the momentum transfer range 0.006<q<0.156 used for analysis (q=4πsinθ/λ, where 2θis the scattering angle andλis the wavelength). (d) Guinier plot for the low-qregion of the SAXS data. Linear agreement of the Guinier equation (red line) with the experimental data (blue crosses) is confirmed by low residuals (red dots) within the boundaries indicated by the arrow, enabling estimation of the radius of gyration,Rg. (e) Inter-atomic pairwise distribution function,P(r), calculated by GNOM. Data were automatically truncated toqmax≈0.16 according to the 8/Rglimit rule forab initiomodelling by DAMMIF. TheP(r) function smoothly approaches zero atDmax=158.1 Å. (f) Theoretical scattering curve (red line) for 1 of 20ab initiomodels generated by DAMMIF, fitted to the experimental data (green crosses). All 20 models were superimposed, averaged and filtered by DAMAVER to generate the final model used for envelope generation inaandb. The mean normalized spatial discrepancy (NSD) for the 20 aligned models was 0.619±0.048, and one model was omitted from averaging as an outlier. Figure 8: SAXS analysis of the HerA–NurA complex. ( a ) and ( b ) lateral and axial views, respectively, of the molecular envelope generated by ab initio SAXS modelling, with crystallographic models of HerA (PDB code: 4D2I) and NurA (PDB code: 2YGK) manually docked in it. The axial view is clipped at the level of the ATPase domains of the HerA hexamer, to visualize the pore-like cavity present in the SAXS envelope, which defines the position of HerA within the map. ( c ) Experimental SAXS curve for the HerA–NurA complex, in the momentum transfer range 0.006< q <0.156 used for analysis ( q =4 π sin θ / λ , where 2 θ is the scattering angle and λ is the wavelength). ( d ) Guinier plot for the low- q region of the SAXS data. Linear agreement of the Guinier equation (red line) with the experimental data (blue crosses) is confirmed by low residuals (red dots) within the boundaries indicated by the arrow, enabling estimation of the radius of gyration, R g . ( e ) Inter-atomic pairwise distribution function, P ( r ), calculated by GNOM. Data were automatically truncated to q max ≈0.16 according to the 8/ R g limit rule for ab initio modelling by DAMMIF. The P ( r ) function smoothly approaches zero at D max =158.1 Å. ( f ) Theoretical scattering curve (red line) for 1 of 20 ab initio models generated by DAMMIF, fitted to the experimental data (green crosses). All 20 models were superimposed, averaged and filtered by DAMAVER to generate the final model used for envelope generation in a and b . The mean normalized spatial discrepancy (NSD) for the 20 aligned models was 0.619±0.048, and one model was omitted from averaging as an outlier. Full size image Ring-shaped multimeric ATPases regulate a wide variety of crucial biological processes such as DNA replication, transcription and repair in cellular and viral systems [1] , [3] , [4] , [43] , [44] . In all cases, the energy liberated from NTP binding and hydrolysis triggers conformational changes that result in mechanical work on the substrate. Similarly, the hexameric ring of the archaeal HerA ATPase harnesses the energy generated from nucleotide hydrolysis to translocate the HerA–NurA complex along DNA substrates [14] , [19] , [21] . To date, our understanding of DNA-end processing in preparation for DNA repair is restricted by our limited structural and mechanistic insight into the helicase–nuclease systems that are predisposed to this task. We have focused our attention on the archaeal HerA–NurA helicase–nuclease complex, which is encoded together with the Mre11–Rad50 complex within a conserved operon of thermophilic archaea [7] , [14] , [17] . Recent evidence shows that DNA-end processing in this archaeal system is substantially different from the established paradigms in the field, such as the bacterial RecBCD, AddAB or AdnAB complexes [24] , [45] , [46] . When taken together, the data presented here lead us to propose a possible mechanism for DNA-end processing by the HerA–NurA complex ( Fig. 9a–d ). Mutagenesis mapping of the reciprocal interaction surfaces for nuclease and helicase ( Fig. 2b ) [16] , and the SAXS analysis of the HerA–NurA complex are compatible with a concentric arrangement of the NurA toroid with the HAS domain ‘crown’ of the HerA ring ( Fig. 8d ; Supplementary Fig. 7 ). Docking of these two annular components would form a coaxial structure, able to thread the DNA substrate through the HerA motor and towards the NurA nuclease. We surmise that DNA would enter the HerA ring via the positively charged face formed by the helix bundle domains, leading to a central channel capable of accommodating up to three turns of B-form dsDNA ( Figs 1f and 9a ). As the DNA substrate exits the HerA channel, it would then be processed by the dimeric NurA nuclease. Since the NurA toroid is too narrow to accommodate B-form dsDNA [16] , the dimeric nuclease would act as a molecular ‘ploughshare’ [23] by melting the DNA duplex and guiding each strand towards its two active sites. High-affinity binding of the single-stranded DNA by NurA [16] is likely to reduce substrate slippage, and enhance processive translocation. Similarly, the E1 papillomavirus helicase has been reported to utilize an analogous, although integral, DNA-binding domain to enhance DNA unwinding, by preventing unproductive sliding [47] . 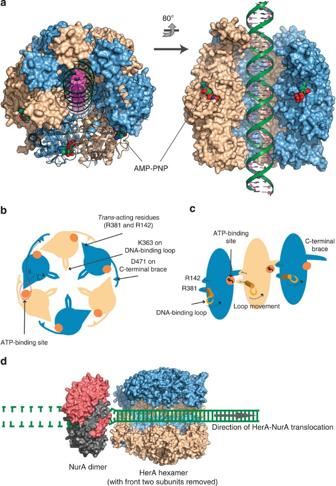Figure 9: A model for dsDNA processing by the HerA–NurA complex. (a) Forty bp dsDNA modelled into the DNA-binding channel of the HerA hexamer, coloured as inFig. 1c. AMP-PNP molecules are shown as spacefill models. Left: top-down view of the HerA hexamer tilted slightly from the vertical position, with four adjacent protomers shown in surface representation and two shown as ribbons. Right: side-view of the HerA hexamer (HAS barrels at the top) with two front protomers omitted. Modelled dsDNA is threaded through the DNA-binding channel of HerA. Models are generated using PyMOL57. (b) Schematic representation of the HerA hexameric ring viewed in the plane of DNA binding. Alternating subunits are coloured in light blue and wheat, respectively. The nucleotide-binding sites, indicated by orange circles, interact intranswith the adjacent subunit via the arginine residues R142 and R381. The putative DNA-binding loops are indicated within the central cavity. The C-terminal ‘brace’ is also presented. The conserved D471 residue on this extension interacts with thetrans-acting R142 residue of the neighbouring subunit. Movements of the R381trans-acting arginine finger will likely translate to the DNA-binding loops and coordinate translocation (i), while communication between the subunits might be regulated by the D471 brace aspartate (ii). (c) Cutaway representation of three HerA subunits, viewed perpendicular to the plane of DNA binding. The association of the D471 C-terminal brace aspartate with the R142trans-acting arginine is also illustrated. (d) A model for how HerA and NurA might cooperate to process DNA ends. HerA (PDB ID 4D2I) is viewed from the side, with two subunits removed to reveal the DNA-binding channel. Interaction with dimeric NurA (red and grey, PDB ID 2YGK) is mediated via the alpha-helical extensions at the N-terminal HAS barrels of HerA, and reciprocal hydrophobic surfaces on the NurA annulus16. Double-stranded DNA is channelled through HerA and unwound by the ploughshare action of NurA. In the model, both DNA strands are engaged by the NurA dimer, resulting in wholesale degradation of the substrate. Figure 9: A model for dsDNA processing by the HerA–NurA complex. ( a ) Forty bp dsDNA modelled into the DNA-binding channel of the HerA hexamer, coloured as in Fig. 1c . AMP-PNP molecules are shown as spacefill models. Left: top-down view of the HerA hexamer tilted slightly from the vertical position, with four adjacent protomers shown in surface representation and two shown as ribbons. Right: side-view of the HerA hexamer (HAS barrels at the top) with two front protomers omitted. Modelled dsDNA is threaded through the DNA-binding channel of HerA. Models are generated using PyMOL [57] . ( b ) Schematic representation of the HerA hexameric ring viewed in the plane of DNA binding. Alternating subunits are coloured in light blue and wheat, respectively. The nucleotide-binding sites, indicated by orange circles, interact in trans with the adjacent subunit via the arginine residues R142 and R381. The putative DNA-binding loops are indicated within the central cavity. The C-terminal ‘brace’ is also presented. The conserved D471 residue on this extension interacts with the trans -acting R142 residue of the neighbouring subunit. Movements of the R381 trans -acting arginine finger will likely translate to the DNA-binding loops and coordinate translocation (i), while communication between the subunits might be regulated by the D471 brace aspartate (ii). ( c ) Cutaway representation of three HerA subunits, viewed perpendicular to the plane of DNA binding. The association of the D471 C-terminal brace aspartate with the R142 trans -acting arginine is also illustrated. ( d ) A model for how HerA and NurA might cooperate to process DNA ends. HerA (PDB ID 4D2I) is viewed from the side, with two subunits removed to reveal the DNA-binding channel. Interaction with dimeric NurA (red and grey, PDB ID 2YGK) is mediated via the alpha-helical extensions at the N-terminal HAS barrels of HerA, and reciprocal hydrophobic surfaces on the NurA annulus [16] . Double-stranded DNA is channelled through HerA and unwound by the ploughshare action of NurA. In the model, both DNA strands are engaged by the NurA dimer, resulting in wholesale degradation of the substrate. Full size image It should be noted that the HerA planar ring observed in the AMP-PNP-bound structure might undergo conformational changes during DNA translocation. In other ring-shaped multimeric ATPases, catalytic activity is driven by an ordered series of events at the nucleotide-binding sites, alternating between ATP-bound, adenosine diphosphate-bound and empty states. This often coincides with the ‘staircasing’ of the DNA-binding loops, or the protomers themselves, to match the pitch of the sugar–phosphate backbone of the DNA [31] , [37] , [38] . In other oligomeric motor protein systems, movements of substrate-binding loops are associated with occupancy and the hydrolysis state of NTP at the nucleotide-binding site, and thus mediate the conversion of chemical energy into mechanical work [31] , [36] , [37] , [39] , [48] . Indeed, DNA-binding loop movement in the P4 hexameric bacteriophage ϕ12 ATPase has also been associated with trans -acting arginine finger positioning [36] . In the HerA hexamer, the proximity of the equivalent R381 trans -acting arginine to the putative DNA-binding loop, harbouring K363 ( Fig. 6 ), suggests that structural changes at the ATP-binding site are transmitted to the substrate-binding channel. Thus, local changes in the positioning of R381, as a result of ATP binding, hydrolysis and release, could result in DNA-binding loop movement, and substrate translocation, similar to reported mechanisms in other multimeric ATPases [1] , [3] , [4] , [10] , [12] ( Fig. 9b,c ). The C-terminal brace observed in the HerA structure is critical for DNA processing by the HerA–NurA complex. An analogous C-terminal brace has been previously visualized at low resolution by SAXS in the papillomavirus E1 helicase, and has been shown to maintain multimeric assembly [28] . In HerA, this brace also appears to regulate the catalytic events at the ATP-binding sites of the hexamer. The conserved brace aspartate 471 forms a salt bridge with the R142 trans -acting arginine from the adjacent subunit ( Figs 3a and 9b,c ). Formation of this salt bridge is likely to dissipate the negative charge on the arginine residue, reducing catalytic potential. Indeed, a D471A mutant exhibits increased ATP turnover, although it is unable to process DNA efficiently ( Fig. 4a,b ). The brace therefore appears to play a role in coupling the chemical events at the catalytic sites into mechanical motion along the DNA. It is tempting to speculate that the C-terminal brace may act as a molecular ‘timing-belt’ to ensure an ordered and sequential propagation of ATP hydrolysis during directional DNA translocation ( Fig. 9b,c ). The R142–D471 association also seems to regulate the ATPase activity of the HerA–NurA complex in response to substrate engagement. Nucleotide turnover in the WT complex is strictly dependent upon DNA binding and is modulated by DNA end-type: overhang substrates elicit only half the level of hydrolysis generated by blunt-ended molecules. Intriguingly, an R142A mutation alleviates this discrepancy by approximately doubling ATP turnover on overhang DNA ( Fig. 4a ). Furthermore, the R142A–D471A mutant is competent to hydrolyse ATP even in the absence of a substrate ( Fig. 4a ). We therefore propose that the R142–D471 interaction captured in our structure might exclude the second arginine finger (R381) from optimal positioning at the active site, until dsDNA is engaged. Our study has revealed the first crystallographic structure of the HerA hexameric ATPase. This completes our structural knowledge of the four individual components of the minimal archaeal end-resection apparatus [19] encoded by the Mre11–Rad50 operon [16] , [18] , [49] , [50] , [51] . Clearly, additional structural and functional studies will be required to elucidate the precise mechanisms that underpin translocation and substrate processing by the HerA–NurA complex. In particular, it remains uncertain how DNA end-resection might be regulated to generate the 3′ single-stranded tails required for HR. It is also unknown how the Mre11–Rad50 DNA repair complex, conserved in eukaryotes and archaea, is involved in the recruitment, or modulation, of the HerA–NurA complex. Future analyses using archaeal models should provide us with new insights into the mechanisms that drive HerA and other multimeric ring-shaped translocases. In addition, these studies should improve our understanding of the helicase–nuclease systems that regulate DNA end-resection, a process essential for HR-mediated DNA repair in all domains of life. Protein purification Untagged native herA and nurA open-reading frames cloned into the pET30 expression vector were purified as described previously [16] . Briefly, cell lysates were heat-clarified and soluble proteins were subsequently purified by affinity chromatography, using a Hi-Trap heparin column and size-exclusion chromatography over a Superdex 200 16/600 column. Mutant constructs were generated from the WT clones by site-directed mutagenesis (QuikChange, Stratagene). Full details are given in the Supplementary Methods . Crystallization and X-ray structure determination A preliminary, incomplete crystal structure of the HerA hexamer bound to AMP-PNP was determined by multi-wavelength anomalous dispersion using selenomethionine-labelled crystals and refined to a resolution of 3.4 Å. This partial structure was then used as a molecular replacement search model for a native data set, ultimately leading to a complete structure refined to 2.85 Å. Full details of crystallization, structure determination and subsequent refinement are given in the Supplementary Methods . Coordinates and structure factors have been deposited in the Protein Data Bank under entry ID 4D2I. Size-exclusion chromatography (analytical gel filtration) Physical interactions between the native NurA protein and either native or mutant HerA proteins were examined by size-exclusion chromatography using an analytical S200 HR 10/300 column (GE Healthcare) as described previously [16] . HerA–NurA complexes were formed at 60 °C, prior to the gel filtration analysis. Further experimental details are described in the Supplementary Methods . Combined HerA–NurA DNA unwinding and nuclease assays The catalytic activity of the native HerA–NurA complex, and also the mutant HerA proteins in complex with native NurA, was examined in a combined DNA-unwinding and digestion assay on a linear 5.5-kb dsDNA substrate (DNA destruction assay). Briefly, 2.5 μM of the HerA hexamer and 2.5 μM NurA dimer were mixed at 60 °C for 20 min to form the complex, before addition of the DNA substrate at 1.25 nM. Reactions were terminated with 0.4% SDS and 0.15 mg ml −1 proteinase K. Products were resolved on a 0.8% agarose gel and visualized with ethidium bromide stain. Further experimental details are described in the Supplementary Methods . DNA-unwinding (helicase) reactions DNA-unwinding reactions, using the D58A nuclease inactive NurA protein [16] . WT or mutant hexameric HerA (0.5 μM) and 0.5 μM dimeric D58A NurA were preincubated at 60 °C for 20 min before addition of a 10-nM 32 P-labelled dsDNA substrate and incubated at 60 °C for 30 min. Reactions were terminated by the addition of 20 μl stop buffer (100 mM EDTA, 0.5% SDS, 0.1 % bromophenol blue and 50% glycerol), and separated on 12% SDS–polyacrylamide gel electrophoresis in 1 × TBE (Tris, Borate, EDTA), 0.2% SDS at 7.5 V cm −1 . Gels were dried and results were visualized by phosphoimaging (GE Healthcare Typhoon system). Further experimental details are described in the Supplementary Methods . ATPase methods The turnover of ATP by mutant HerA–NurA complexes was determined as previously described in earlier work [16] , utilizing a proprietary malachite dye kit (P i ColorLock Gold—Innova Biosciences) to monitor the release of inorganic phosphate (P i ). Variations to these methods are described in the Supplementary Data . Triplex displacement assays Triplex displacement assays were based on the method of Firman and Szczelkun [35] , but using a SwaI linearized form of the plasmid pLKS5, positioning the 22 nucleotide triplex-forming oligo (TFO) centrally within the 7,500-bp vector. The TFO was end labelled with γ- 32 P using polynucleotide kinase. Triplexes were formed as previously described [16] , [35] . WT or mutant HerA and D58A NurA proteins were preincubated in reaction buffer (25 mM MES, 50 mM NaCl, 10 mM MgCl2, 0.5 mM spermidine and 3 mM ATP, pH 5.5) at 60 °C for 30 min and then cooled to 50 °C. Triplex (5 nM) was added to the HerA–NurA complex and incubated at 50 °C for appropriate time. Reactions were terminated by cooling on ice and addition of 6 × glycerol loading buffer (30% glycerol, 20 mM Tris pH 8, 0.25% bromophenol blue and 0.6% SDS). Products were resolved on 1% agarose gels in 40 mM tris-acetate, 5 mM sodium acetate, 1 mM MgCl 2 , pH 5.5 buffer at 120 V for 2.5 h at 4 °C, and viewed by phosphoimaging. Further experimental details are described in the Supplementary Methods . Helicase complementation assays (mutant-doping assays) Native and catalytically inactivated (K154A) HerA were mixed together at the ratios indicated and incubated at 60 °C for 20 min, to permit the formation of hybrid hexamers. Dimeric D58A (nuclease inactivated) NurA was then added and the reaction incubated for a further 20 min at 60 °C to allow the formation of the HerA–D58ANurA complex. The hybrid complexes were then used in the helicase assays as described above. Further experimental details are provided in the Supplementary Methods . Small-angle X-ray scattering SAXS data were collected at the SWING beamline of the SOLEIL synchrotron (Gif-sur-Yvette, France) using a robotic sample changer and an Agilent HPLC-coupled SAXS cell [52] , [53] . Prior to sample loading, 60 μl of the HerA–NurA complex (using HerA harbouring both M51L and M82L mutations, and NurAD58A) were formed by heating individual components together at 60 °C for 20 min, at a final concentration of 14.2 μM (assuming a 6:2 HerA:NurA stoichiometry), with a fourfold excess of NurAD58A dimer, in the presence of 0.2 mM ATP and 1 mM MgCl 2 . Approximately 50 μl protein was injected into the SAXS flow-through cell at a flow rate of 150 μl min −1 via a size-exclusion chromatography column (GE Superdex 200 Increase 3.2/300) pre-equilibrated with SAXS buffer (20 mM Hepes pH 7.0, 300 mM NaCl, 5% v/v glycerol, 0.2 mM ATP and 1 mM MgCl 2 ). The quartz capillary cell (1.5 mm diameter, 10 μm wall thickness) was thermostated to 288 K during data collection. Both cell and detector (a 17 × 17 cm 2 low-noise Aviex CCD) were housed in a vacuum chamber, with a sample-detector distance of 1.786 m. Approximately 250 frames of scattering data were collected at a wavelength ( λ ) of 1.022 Å during sample elution, with 1.5-s frame duration and 0.5-s dead time between frames. A dedicated in-house application (‘FOXTROT’) was used to average frames across the elution peak of the complex and subtract buffer scattering. Averaged SAXS data were subsequently processed by components of the ATSAS package [53] . Briefly, in PRIMUS the forward scattering I (0) and the radius of gyration R g were evaluated using the Guinier approximation: for small angles ( q <1.3/ R g ), I ( q )= I (0) exp(−(1/3)( qR g ) 2 ). The indirect transform package GNOM confirmed these parameters from the entire data range and calculated the pair-distance distribution function P ( r ), enabling estimation of the maximum particle dimension, D max . The ab initio modelling program DAMMIF was used for low-resolution shape analysis, with 20 independent models generated in the ‘slow’ mode and subsequently averaged and filtered by DAMAVER. The latter program also yielded a value of normalized spatial discrepancy, used to determine similarities between different models and identify outliers. A molecular envelope was generated from the filtered averaged bead model using the pdb2vol component of the Situs package [54] . Crystallographic models of HerA (PDB code: 4D2I) and NurA (PDB code: 2YGK [16] ) were manually docked into the molecular envelope and visualized using the UCSF Chimera package [55] , [56] . How to cite this article: Rzechorzek, N. J. et al. Structure of the hexameric HerA ATPase reveals a mechanism of translocation-coupled DNA-end processing in archaea. Nat. Commun. 5:5506 doi: 10.1038/ncomms6506 (2014). Accession codes : The coordinates and structure factors of the S. solfataricus HerA crystal structure have been deposited in the Protein Data Bank under accession code 4D2I .